Muscarinic acetylcholine receptor M3 modulates odorant receptor activity via inhibition of β-arrestin-2 recruitment The olfactory system in rodents serves a critical function in social, reproductive and survival behaviours. Processing of chemosensory signals in the brain is dynamically regulated in part by an animal’s physiological state. We previously reported that type 3 muscarinic acetylcholine receptors (M3-Rs) physically interact with odorant receptors (ORs) to promote odour-induced responses in a heterologous expression system. However, it is not known how M3-Rs affect the ability of olfactory sensory neurons (OSNs) to respond to odours. Here, we show that an M3-R antagonist attenuates odour-induced responses in OSNs from wild-type, but not M3-R-null, mice. Using a novel molecular assay, we demonstrate that the activation of M3-Rs inhibits the recruitment of β-arrestin-2 to ORs, resulting in a potentiation of odour-induced responses in OSNs. These results suggest a role for acetylcholine in modulating olfactory processing at the initial stages of signal transduction in the olfactory system. The olfactory system allows animals to interact with their environment and respond to signals of predation, mating and feeding. The type of olfactory information animals require drastically differs depending on their behavioural state, for example, during hunting, mate-seeking or sleeping. While a number of recent studies have examined the behavioural state regulation of olfactory processing at higher-level information processing centres in the brain, little is known as to how olfactory processing is regulated by physiological state at the level of olfactory sensory neurons (OSNs), partly owing to the complexity and diversity of odorant receptor (OR)-ligand coding. Odour detection is initiated by the activation of OR proteins located at the cilia of OSNs in the olfactory epithelium (OE). ORs make up the largest family of the seven transmembrane, G-protein-coupled receptor (GPCR) superfamily, encompassing ~400 and 1,200 OR proteins in human and mouse, respectively [1] , [2] , [3] . Odour recognition in mammals is integrative, depending on a constellation of receptor–ligand interactions that activate a repertoire of ORs expressed by defined subsets of OSNs [4] . The activated ORs lead to increased intracellular cAMP levels via the sequential activation of olfactory G-protein (Golf) [5] and type III adenylyl cyclase (ACIII) [6] . Elevated cAMP levels lead to the opening of cyclic nucleotide-gated channels [7] and influx of cations including Ca 2+ . The cation influx, together with the efflux of Cl − by a Ca 2+ -activated Cl − channel results in a depolarization in OSNs, which leads to further Ca 2+ influx via voltage-gated Ca 2+ channels and ultimately triggers action potentials that transmit odour information downstream to the olfactory bulb [8] . On the other hand, β-arrestin-2 inhibits OR activation [9] , [10] , presumably by competing with G-protein for GPCR binding [11] to mediate receptor deactivation and internalization [12] . In addition, β-arrestins function as scaffolds and recruit signalling molecules that mediate specific pathways including mitogen-activated protein (MAP) kinases on their own [13] . It is not clear how β-arrestin recruitment is regulated in the OSNs. The OE is a highly specialized tissue that receives extensive innervation from parasympathetic nerve endings that release acetylcholine [14] , [15] , [16] . Cholinergic microvillous cells distributed throughout the OE may provide an alternative or additional source of acetylcholine [17] . Functional studies in amphibian OSNs showed that acetylcholine receptor agonists potentiated odour responses and increased the excitability of OSNs [18] , [19] , and that antagonists of muscarinic acetylcholine receptors resulted in the opposite effects [20] . We previously reported that the type 3 muscarinic acetylcholine receptor (M3-R) physically interacts with ORs to promote odour-induced responses in vitro and showed that M3-selective antagonists attenuated odour-induced Ca 2+ responses in dissociated OSNs [21] . On the other hand, acetylcholine has been shown to suppress Ca 2+ increases in some OSNs induced by an adenylyl cyclase activator forskolin [17] . Thus, it remains unclear whether and how acetylcholine potentiates OSN activity. In the present study, we examine the role of M3-R in regulating odour responses in OSNs using a combination of pharmacological and genetic approaches. We show that OSNs from M3-R knockout (KO) mice exhibit decreased odour response amplitudes, are less likely to respond to odour stimulation and do not show a reduction in odour responses in the presence of darifenacin as compared with OSNs from wild-type (WT) mice. Moreover, application of the muscarinic agonist carbachol or the physiological M3-R ligand acetylcholine resulted in increased odour-induced responses in OSNs. To identify the mechanism, we used a novel β-arrestin-2 recruitment assay for ORs expressed in heterologous cells to show that M3-R inhibits β-arrestin-2 recruitment in ORs in an activity-dependent manner. In addition, β-arrestin-2 deficiencies attenuate the potentiation of OR-mediated cAMP responses by M3-R. Interestingly, these effects cannot be explained by competition for β-arrestin-2 between M3-R and ORs. Finally, we show that the third intracellular loop (i3) of M3-R is important for inhibiting OR/β-arrestin-2 interactions. Together, our results demonstrate that M3-Rs modulate OR activity by regulating β-arrestin-2 recruitment, thus revealing a novel mechanism for acetylcholine in regulating olfactory sensory processing at the peripheral level. M3-Rs are expressed in the cilia layer of the OE We have previously shown that the M3-R protein [22] is expressed in the cilia of OSNs and that M3-R mRNA transcripts are detectable in OSN somata [21] . However, it was recently reported that the M3-R protein was expressed by the supporting cells rather than primarily in OSNs [17] . In order to validate and characterize the expression pattern of M3-Rs, we performed immunostaining of the OSN cilia with the M3-R antibody in WT (or M3-R +/+ ) and M3-R KO (or M3-R −/− ) mice [23] . Dolichos biflorus agglutinin, a plant lectin that labels a subset of OSNs [24] , [25] , was used to stain the cilia layer. We detected robust M3-R staining in the OSN cilia of WT animals ( Fig. 1a ; n =8 sections from four animals). As expected, OSN cilia obtained from M3-R KO mice did not show detectable M3-R staining ( Fig. 1b ; n =6 sections from two animals), supporting our previous find that M3-Rs are specifically expressed in OSNs. In addition, we noted that the gross anatomy of the OE as well as the cilia morphology in whole-mount OE attached to the septal wall from M3-R KO mice is indistinguishable from that of WT littermates ( Supplementary Fig. 1 ; n =4 epithelial preparations from two animals for each condition). These results suggest that genetic ablation of M3-Rs does not affect the anatomical development or organization of OSNs in the OE. 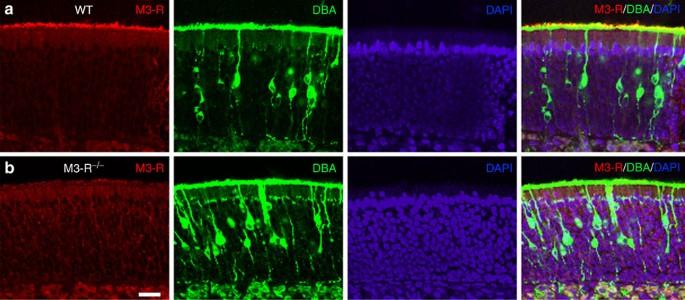Figure 1: M3-R antibody stains the cilia layer of the OE in WT but not in M3-R KO mice. Coronal sections of the nose were stained with the M3-R antibody (red), Dolichos biflorus agglutinin (DBA; green) and 4′,6-diamidino-2-phenylindole (blue) in WT (a) and M3-R KO mice (b). Confocal images were taken at a single plane withzstep=1 μm. Scale bar=20 μm and applies to all panels. Figure 1: M3-R antibody stains the cilia layer of the OE in WT but not in M3-R KO mice. Coronal sections of the nose were stained with the M3-R antibody (red), Dolichos biflorus agglutinin (DBA; green) and 4′,6-diamidino-2-phenylindole (blue) in WT ( a ) and M3-R KO mice ( b ). Confocal images were taken at a single plane with z step=1 μm. Scale bar=20 μm and applies to all panels. Full size image M3-Rs modulate odorant-induced responses of OSNs We previously showed that acutely dissociated OSNs from WT mice exhibit attenuated odour-mediated Ca 2+ responses in the presence of M3-R-preferring antagonist darifenacin [21] . If the modulation of OSN activation by darifenacin is attributable to M3-R-related inhibition, then darifenacin is expected to have no effect in M3-R KO mice. To test this, we compared odour-induced Ca 2+ responses of dissociated OSNs derived from M3-R −/− mice and M3-R +/+ littermates in response to a mixture of 10 odorants with or without 0.1 μM darifenacin (see Methods section). While odour responses were significantly attenuated by darifenacin in M3-R +/+ OSNs ( Fig. 2a,b , P <0.0001, two-tailed paired t -test, n =36 pairs), darifenacin had no significant effect on odour-induced responses in M3-R −/− OSNs ( Fig. 2c,d , P =0.4183, two-tailed paired t -test, n =62 pairs). These results demonstrate that darifenacin inhibits odour-mediated Ca 2+ responses of OSNs in an M3-R-dependent manner. 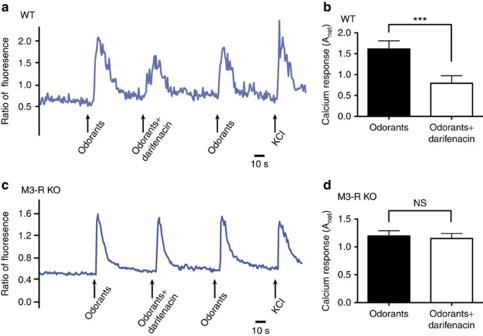Figure 2: Darifenacin attenuates odour-induced Ca2+signals of dissociated OSNs in WT but not in M3-R KO mice. (a) A single cell from an M3-R+/+mouse was stimulated by a mixture of 10 odorants each at a concentration of 10 μM with or without 0.1 μM darifenacin. The Ca2+signals were monitored as fluorometric ratios (Fluo-4/Fura-red). KCl serves as a positive control. (b) Darifenacin significantly reduced odour-induced Ca2+signals (two-tailed pairedt-test;n=36 pairs). (c) A single cell from an M3-R−/−mouse was stimulated by a mixture of 10 odorants each at 10 μM with or without 0.1 μM darifenacin. (d) Darifenacin failed to attenuate odour-mediated responses of OSNs from M3-R−/−mice (two-tailed pairedt-test,n=62 pairs). ***P<0.001. NS, not significant. Figure 2: Darifenacin attenuates odour-induced Ca 2+ signals of dissociated OSNs in WT but not in M3-R KO mice. ( a ) A single cell from an M3-R +/+ mouse was stimulated by a mixture of 10 odorants each at a concentration of 10 μM with or without 0.1 μM darifenacin. The Ca 2+ signals were monitored as fluorometric ratios (Fluo-4/Fura-red). KCl serves as a positive control. ( b ) Darifenacin significantly reduced odour-induced Ca 2+ signals (two-tailed paired t -test; n =36 pairs). ( c ) A single cell from an M3-R −/− mouse was stimulated by a mixture of 10 odorants each at 10 μM with or without 0.1 μM darifenacin. ( d ) Darifenacin failed to attenuate odour-mediated responses of OSNs from M3-R −/− mice (two-tailed paired t -test, n =62 pairs). *** P <0.001. NS, not significant. Full size image While Ca 2+ imaging of dissociated OSNs can simultaneously assess the stimulated response profiles of dozens of OSNs, it is an indirect measure of OSN activation, since Ca 2+ influx occurs several steps downstream from OR activation, which is where M3-Rs are expected to interact with ORs. Another concern is that enzymatic and mechanical OSN dissociation may alter the physiological activity of OSNs. To more directly investigate how M3-Rs modulate OR activation, we performed perforated patch-clamp recordings on the dendritic knobs of in situ OSNs from intact OE [26] . Under voltage-clamp mode, brief puffs of an odorant mixture (19 odorants at equal molar concentration of 100 μM; see Methods section for details) elicited inward currents in 72.5% (50 out of 69) of randomly chosen OSNs from WT animals (including WT C57BL/6 mice and M3-R +/+ littermate controls, see below). Out of the 50 odour-responsive cells (defined as when odour-induced currents >5 pA), we were able to measure the responses induced by the odorant mixture with or without 0.1 μM darifenacin in 41 cells ( Fig. 3 ) by alternating between two barrels of the puffing pipette (odorants or odorants+darifenacin; see Methods section). In a single cell, we performed multiple (typically 3–4) rounds of stimulation and averaged the peak currents from all trials with identical stimuli. 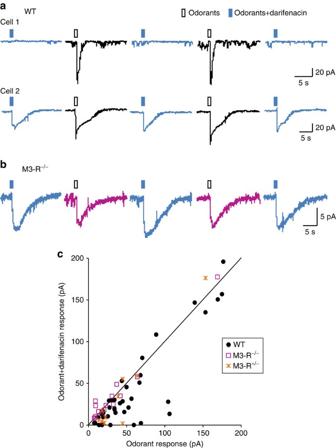Figure 3: Darifenacin attenuates odour-induced electrical responses of OSNs in WT but not in M3-R KO mice. Individual OSNs were alternately stimulated by puffs of odorants (100 μM, hollow rectangles) or odors plus darifenacin (0.1 μM, filled rectangles) under voltage-clamp mode. (a) Darifenacin completely (cell 1) or partially (cell 2) blocks odour-induced responses in WT OSNs. (b) Darifenacin does not attenuate odor-induced responses in OSNs from M3-R KO mice. (c) The peak current induced by odorants+darifenacin (averaged from all trials in each cell) is plotted against that induced by odorants alone. The identity line represents equal responses from the two stimuli. The holding potential was −65 mV for all neurons. Figure 3: Darifenacin attenuates odour-induced electrical responses of OSNs in WT but not in M3-R KO mice. Individual OSNs were alternately stimulated by puffs of odorants (100 μM, hollow rectangles) or odors plus darifenacin (0.1 μM, filled rectangles) under voltage-clamp mode. ( a ) Darifenacin completely (cell 1) or partially (cell 2) blocks odour-induced responses in WT OSNs. ( b ) Darifenacin does not attenuate odor-induced responses in OSNs from M3-R KO mice. ( c ) The peak current induced by odorants+darifenacin (averaged from all trials in each cell) is plotted against that induced by odorants alone. The identity line represents equal responses from the two stimuli. The holding potential was −65 mV for all neurons. Full size image We observed that coadministration of 0.1 μM darifenacin either abolished ( Fig. 3a , cell 1) or reduced ( Fig. 3a , cell 2) odour-induced responses. The peak currents were significantly reduced in the presence of darifenacin (odorants: 67.4±10.9 pA and odorants+darifenacin: 52.2±11.1 pA, n =41, P <0.0002 in two-tailed, paired t -test). To compare the effects of darifenacin across all cells, we plotted the peak current induced by odorants+darifenacin versus that by odorants alone for each of the 41 cells ( Fig. 3c ). We observed that most points fell below the identity line y = x , indicating that the effects of darifenacin were largely independent of the cell-to-cell variations in odour responses. In summary, our electrophysiological results demonstrate that a selective M3-R antagonist reduces odour responses of OSNs from WT animals, consistent with our in vitro and Ca 2+ -imaging data [21] ( Fig. 2 ). Given that M3-R antagonism inhibits OR activation, we next asked whether activation of M3-Rs would potentiate odour responses in OSNs. We tested the effects of cholinergic agonists on odour responses by patch-clamp recordings in an independent set of OSNs in WT animals ( Fig. 4 ). A total of 30 odour-responsive cells were tested with 1 μM carbachol (odorants+Ringer’s solution: 25.2±3.2 pA and odorants+carbachol at 1 μM: 42.5±5.3 pA, n =30, P <0.0002 in two-tailed, paired t -test). Among these 30 cells, 17 cells were also tested with 0.1 μM carbachol (odorants+Ringer’s: 22.7±5.1 pA and odorants+carbachol at 0.1 μM: 47.5±9.8 pA, n =17, P =0.0012 in paired t -test), and 15 cells were also stimulated with 1 μM acetylcholine (odorants+Ringer’s: 24.8±5.6 pA and odorants+ACh: 48.6±10.8 pA, n =15, P =0.0050 in paired t -test). The raw data from one OSN tested with all three agonist solutions are shown in Fig. 4a . For each cell, we plotted the peak current induced by odorants+agonist against that induced by odorants+Ringer’s solution ( Fig. 4b ). Most data points lie above the identity line, indicating that cholinergic agonists enhance odour responses in OSNs. 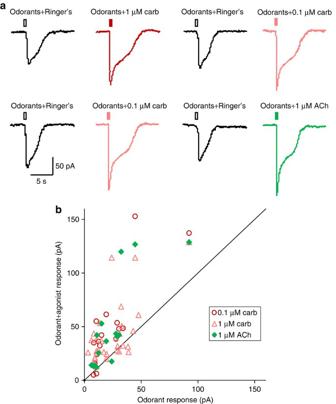Figure 4: M3-R agonists enhance odour-induced responses of OSNs. (a) A single OSN was alternately stimulated by puffs of odorants+Ringer’s solution (hollow rectangles in black), odorants+carbachol (carb) at 1 μM (filled rectangle in red) or 0.1 μM (filled rectangle in pink), or odorants+acetylcholine (ACh) at 1 μM (filled rectangles in green) under voltage-clamp mode. All odorants were presented at a concentration of 100 μM. The two rows are sequential recordings from the same cell. (b) The peak current induced by odorants+agonist (averaged from all trials in each cell) is plotted against that induced by odorants+Ringer’s solution. The identity line represents equal responses from the two stimuli. The holding potential was −65 mV for all neurons. Figure 4: M3-R agonists enhance odour-induced responses of OSNs. ( a ) A single OSN was alternately stimulated by puffs of odorants+Ringer’s solution (hollow rectangles in black), odorants+carbachol (carb) at 1 μM (filled rectangle in red) or 0.1 μM (filled rectangle in pink), or odorants+acetylcholine (ACh) at 1 μM (filled rectangles in green) under voltage-clamp mode. All odorants were presented at a concentration of 100 μM. The two rows are sequential recordings from the same cell. ( b ) The peak current induced by odorants+agonist (averaged from all trials in each cell) is plotted against that induced by odorants+Ringer’s solution. The identity line represents equal responses from the two stimuli. The holding potential was −65 mV for all neurons. Full size image To exclude the possibility that darifenacin inhibits OSN responses due to toxicity or nonspecific effects, we compared patch-clamp analysis of OSNs in intact OE from WT (including littermate M3-R +/+ ), heterozygous (HET or M3-R +/− ) and KO (M3-R −/− ) mice. As expected, the responses were not attenuated in the presence of 0.1 μM darifenacin from 14 odour-responsive OSNs in M3-R −/− mice ( Fig. 3b,c ) (odorants: 32.9±11.3 pA and odorants+darfenacin: 35.4±11.6 pA, n =14, P =0.2761 in paired t -test). In the 10 OSNs obtained from heterozygous M3-R +/− mice, we did observe a trend of attenuation in odour responses by darifenacin ( Fig. 3c ), but the effect was not significant (odorants: 43.7±13.2 pA and odorants+darifenacin: 36.5±16.9 pA, n =10, P =0.2276 in paired t -test). These findings confirm that the effects of M3-R antagonism on odour responses are abolished in M3-R −/− mice. Given that M3-R antagonism attenuated odour responses of OSNs in WT animals and that basal expression of M3-Rs without M3-R agonists was sufficient to potentiate OR responses in vitro , we asked whether the loss of M3-R expression would reduce the sensitivity and/or the response amplitude of odour-induced OSN responses. Indeed, the average peak current of odour responses in OSNs from M3-R −/− mice was ~33 pA compared with ~68 pA in WT OSNs recorded under similar conditions ( P =0.0352, two-tailed t -test). More strikingly, the likelihood of an OSN to respond to the odorant mixture stimulation was significantly lower ( P =0.019, Fisher’s exact test) in M3-R −/− mice (18 out of 45 or 40.0% of tested cells) compared with their M3-R +/+ littermates (27 out of 41 or 65.8%), suggesting that the expression of M3-Rs affects the odour response threshold of OSNs. Together, these results constitute the first demonstration that lack of M3-R expression results in functional deficits in mammalian OSNs. The M3-R-activated PLC pathway is not required for OR potentiation Thus far, we have shown that the role of M3-Rs in OR activation is physiologically relevant and consistent with our in vitro observations. However, we have little understanding of the molecular basis by which M3-Rs potentiate OR activation. A number of models could potentially account for the activation and they can be largely divided into the following two categories: (1) the physical interaction of the two receptors promotes odour-induced OR activation; (2) the potentiation is the result of downstream cross talk between OR- and M3-R-mediated PLC-IP3 (Phospholipase C-Inositol triphosphate) signalling, independent of physical interaction ( Fig. 5a ). To test the possibility that M3-R-mediated OR potentiation results from downstream signalling pathways, we exposed HEK293T cells expressing OR-S6, M3-Rs and RTP1S to nonanedioic acid, a potent OR-S6 ligand, in the presence or absence of the PLC inhibitor U73122 (5 μM). We observed no significant differences in the OR-mediated cAMP response with or without application of the PLC inhibitor ( P =0.20; Fig. 5b ), while application of the PLC inhibitor almost completely abolished endoplasmic reticulum Ca 2+ release downstream of the PLC-IP3 pathway ( Fig. 5c ). These results indicate that blocking PLC downstream of the M3-R signalling pathway does not affect the potentiation of OR-mediated cAMP responses by M3-R. 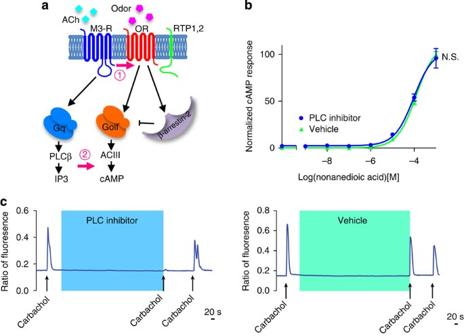Figure 5: Possible mechanisms for M3-R-mediated regulation of OR activation. (a) M3-R could regulate OR activation through (1) the interaction of the two receptors that promotes odour-induced OR activation, or (2) the potentiation is the result of downstream cross talk between OR-mediated cAMP signaling and M3-R-mediated PLC-IP3 signaling, independent of physical interactions. (b) cAMP responses of HEK293T cells expressing OR-S6, M3-R and RTP1S challenged by nonanedioic acid (OR-S6 ligand) in the presence of 5 μM PLC inhibitor U73122 or vehicle DMSO. U73122 showed no effect on OR-S6 response with M3-R coexpression (two-way ANOVA,P=0.20). (c) PLC inhibitor (5 μM) U73122 abolishes the endoplasmic reticulum (ER) Ca2+response, demonstrating effective PLC inhibition. Ach, acetylcholine; NS, not significant. Figure 5: Possible mechanisms for M3-R-mediated regulation of OR activation. ( a ) M3-R could regulate OR activation through (1) the interaction of the two receptors that promotes odour-induced OR activation, or (2) the potentiation is the result of downstream cross talk between OR-mediated cAMP signaling and M3-R-mediated PLC-IP3 signaling, independent of physical interactions. ( b ) cAMP responses of HEK293T cells expressing OR-S6, M3-R and RTP1S challenged by nonanedioic acid (OR-S6 ligand) in the presence of 5 μM PLC inhibitor U73122 or vehicle DMSO. U73122 showed no effect on OR-S6 response with M3-R coexpression (two-way ANOVA, P =0.20). ( c ) PLC inhibitor (5 μM) U73122 abolishes the endoplasmic reticulum (ER) Ca 2+ response, demonstrating effective PLC inhibition. Ach, acetylcholine; NS, not significant. Full size image A quantitative β-arrestin-2 recruitment assay for ORs Another mechanism by which M3-Rs could potentiate OR-mediated G-protein signalling may be via inhibition of alternative signalling, thus leading to increased cAMP release following odour stimulation. Specifically, we hypothesized that M3-Rs inhibit the recruitment of β-arrestin-2 to activated ORs. To test this model, we developed a quantitative and efficient assay to measure OR-mediated β-arrestin-2 recruitment by combining our in vitro OR expression assay [27] with a split-luciferase system [28] ( Fig. 6a ; see Methods section for details). 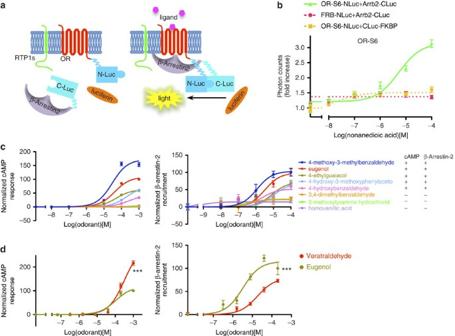Figure 6: β-Arrestin-2 recruitment assay for ORs. (a) An overview. The luciferase gene is split into two fragments (NLuc and CLuc) and fused to the termini of OR and β-arrestin-2. RTP1S enhances the surface expression of many ORs (left). When ligand is present, the OR is activated and recruits β-arrestin-2. The association between the OR and β-arrestin-2 brings the two fragments of luciferase close to each other to form a functional enzyme, resulting in above-background light emission in the presence of luciferin. (b) Dose–response curve of β-arrestin-2 recruitment by a mouse OR, S6, stimulated by its ligand nonanedioic acid. Photon counts were normalized to background emission when no ligand is present to show the fold increase. Dose-dependent light emission was observed when OR-NLuc and Arrb2-CLuc were expressed, but not when either of them was substituted with control protein tagged with corresponding luciferase fragment (FRB-NLuc and CLuc-FKBP). (c) Dose–response curve of cAMP response and β-arrestin-2 recruitment for OR-EG when challenged with various chemicals, and summary of positive and negative responses. (d) Biased signaling towards cAMP pathway of the ligand veratraldehyde, as compared with eugenol.n=3, error bars indicate standard errors. ***P<0.001. Figure 6: β-Arrestin-2 recruitment assay for ORs. ( a ) An overview. The luciferase gene is split into two fragments (NLuc and CLuc) and fused to the termini of OR and β-arrestin-2. RTP1S enhances the surface expression of many ORs (left). When ligand is present, the OR is activated and recruits β-arrestin-2. The association between the OR and β-arrestin-2 brings the two fragments of luciferase close to each other to form a functional enzyme, resulting in above-background light emission in the presence of luciferin. ( b ) Dose–response curve of β-arrestin-2 recruitment by a mouse OR, S6, stimulated by its ligand nonanedioic acid. Photon counts were normalized to background emission when no ligand is present to show the fold increase. Dose-dependent light emission was observed when OR-NLuc and Arrb2-CLuc were expressed, but not when either of them was substituted with control protein tagged with corresponding luciferase fragment (FRB-NLuc and CLuc-FKBP). ( c ) Dose–response curve of cAMP response and β-arrestin-2 recruitment for OR-EG when challenged with various chemicals, and summary of positive and negative responses. ( d ) Biased signaling towards cAMP pathway of the ligand veratraldehyde, as compared with eugenol. n =3, error bars indicate standard errors. *** P <0.001. Full size image In this system, we expressed ORs and β-arrestin-2 tagged with luciferase fragments (OR-S6-NLuc, ~84 kDa and Arrb2-CLuc, ~63 kDa; Supplementary Fig. 2 ) in HEK293T cells along with RTP1S, an accessory protein required for the efficient trafficking of many ORs [27] , [29] , observing that as expected, the cells exhibited increased bioluminescence following nonanedioic acid stimulation in a dose-dependent manner. In contrast, when either OR-NLuc or Arrb2-CLuc was substituted with control proteins tagged with corresponding luciferase fragments (FRP-NLuc and CLuc-FKBP [28] , two proteins known to form a complex in the presence of rapamycin but have no known involvement in olfactory signalling pathways), the dose-dependent response was abolished, indicating that the observed β-arrestin-2 recruitment upon odour stimulation was OR specific ( Fig. 6b ). We also observed dose-dependent β-arrestin-2 recruitment for three additional ORs ( Supplementary Fig. 3 ), and demonstrated that the observed β-arrestin-2 recruitment occurred in a RTP1S-dependent manner for receptors that require RTP1S coexpression for cell-surface trafficking ( Supplementary Fig. 3 ). The tagged ORs showed normal cAMP responses to their cognate ligands and the responses were potentiated by M3-R coexpression ( Supplementary Fig. 4 ). To further demonstrate the specificity of this assay, we measured β-arrestin-2 recruitment to an OR, OR-EG, following stimulation with various chemicals with similar structure to its well-defined ligand, eugenol [30] . The measured β-arrestin-2 recruitment agreed with the cAMP responses for each chemical tested, in that the chemicals that induced cAMP response also led to β-arrestin-2 recruitment ( Fig. 6c ). In addition, we found that one chemical, veratraldehyde, elicited stronger cAMP responses than β-arrestin-2 recruitment ( Fig. 6d ), suggesting that the concept of biased GPCR signalling, in which a ligand preferentially triggers G-protein or β-arrestin-mediated signalling pathways [31] , may be extended to ORs. M3-R specifically inhibits β-arrestin-2 recruitment to ORs Using the in vitro OR-β-arrestin-2 recruitment assay, we tested the hypothesis that M3-R inhibits β-arrestin-2 recruitment to activated ORs. Of the four different ORs tested, we found that M3-R inhibited β-arrestin-2 recruitment in all instances, as compared with the control transmembrane protein CD28 (OR-S6: P =0.01, Olfr62: P =0.03, OR-EG: P <10 −3 and MOR18-2: P <10 −4 ), or another muscarinic receptor M2-R (OR-S6: P <10 −3 , Olfr62: P <10 −4 , OR-EG: P =0.04 and MOR18-2: P <10 −4 ; Fig. 7a ). This result suggests that M3-R inhibits β-arrestin-2 recruitment to ORs and that M3-R functionally associates with ORs to inhibit β-arrestin-2 interaction with ORs to promote OR activation. 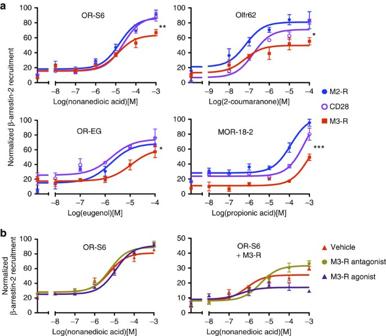Figure 7: M3-R inhibits β-arrestin-2 recruitment to ORs. (a) M3-R inhibits β-arrestin-2 recruitment to the OR. β-Arrestin-2 recruitment of two ORs when different proteins were coexpressed. β-Arrestin-2 recruitment to activated ORs was inhibited when M3-R was coexpressed as compared with the control transmembrane protein CD28 (two-way ANOVA; OR-S6:P=0.01; Olfr62:P=0.03; OR-EG:P<10−3; MOR18-2:P<10−4), or to another muscarinic receptor M2-R (OR-S6:P<10−3; Olfr62:P<10−4; OR-EG:P=0.04; MOR18-2:P<10−4). (b) Activated M3-R inhibits β-arrestin-2 recruitment to the OR. In HEK293T cells coexpressing M3-R, coadministration of M3-R agonist Carbachol (0.1 μM) further decreased β-arrestin-2 recruitment of OR-S6 (P<10−4, two-way ANOVA, right, purple), while coadministration of M3-R antagonist atropine (1 μM) attenuated the block at high odorant concentrations including 100 μM and 1 mM (P<10−4, two-way ANOVA, right, green), as compared with the vehicle DMSO (right, red). These alterations were not observed when M3-R was not coexpressed (P=0.1,P=0.1, two-way ANOVA, left).n=3, error bars indicate standard errors. *P<0.05, **P<0.02, ***P<0.001. Figure 7: M3-R inhibits β-arrestin-2 recruitment to ORs. ( a ) M3-R inhibits β-arrestin-2 recruitment to the OR. β-Arrestin-2 recruitment of two ORs when different proteins were coexpressed. β-Arrestin-2 recruitment to activated ORs was inhibited when M3-R was coexpressed as compared with the control transmembrane protein CD28 (two-way ANOVA; OR-S6: P =0.01; Olfr62: P =0.03; OR-EG: P <10 −3 ; MOR18-2: P <10 −4 ), or to another muscarinic receptor M2-R (OR-S6: P <10 −3 ; Olfr62: P <10 −4 ; OR-EG: P =0.04; MOR18-2: P <10 −4 ). ( b ) Activated M3-R inhibits β-arrestin-2 recruitment to the OR. In HEK293T cells coexpressing M3-R, coadministration of M3-R agonist Carbachol (0.1 μM) further decreased β-arrestin-2 recruitment of OR-S6 ( P <10 −4 , two-way ANOVA, right, purple), while coadministration of M3-R antagonist atropine (1 μM) attenuated the block at high odorant concentrations including 100 μM and 1 mM ( P <10 −4 , two-way ANOVA, right, green), as compared with the vehicle DMSO (right, red). These alterations were not observed when M3-R was not coexpressed ( P =0.1, P =0.1, two-way ANOVA, left). n =3, error bars indicate standard errors. * P <0.05, ** P <0.02, *** P <0.001. Full size image To test this pharmacologically, we coexpressed OR-S6-NLuc, Arrb2-CLuc and RTP1S along with M3-R in HEK293T cells, and stimulated the cells with nonanedioic acid in the presence of either 0.1 μM carbachol (muscarinic agonist) or 1 μM atropine (muscarinic antagonist). As expected, costimulation with carbachol further reduced β-arrestin-2 recruitment to the OR ( P <10 −3 ), while costimulation with atropine led to a significant enhancement of β-arrestin-2 recruitment at high odorant concentrations ( P =0.03, 100 μM and 1 mM nonanedioic acid; Fig. 7b , right). In the absence of M3-Rs, changes in β-arrestin-2 recruitment to ORs were not observed ( Fig. 7b , left), supporting a model in which the activated form of M3-R inhibits β-arrestin-2 recruitment to ORs to promote OR activation. β-arrestin-2 is required for the potentiation of OR responses by M3-R If M3-Rs mainly potentiate cAMP responses of OSNs by inhibiting β-arrestin-2 recruitment, β-arrestin-2 deficiencies should abolish or reduce the effect of M3-Rs. To test this hypothesis, we knocked down the endogenous β-arrestin-2 in HEK293T cells using short interfering RNA (siRNA) [32] , and examined the potentiation of OR-induced cAMP response by M3-R. Depletion of β-arrestin-2 led to a strong potentiation of OR-mediated cAMP response, indicating that a decrease in β-arrestin-2 leads to increased OR activation. As expected, although OR signalling was potentiated by M3-R in cells transfected with control siRNA ( P <10 −4 ; Fig. 8a ), transfection of β-arrestin-2 siRNA abolished the ability of M3-Rs to potentiate OR-mediated cAMP response ( P =0.63). The efficiency of knockdown was confirmed by western blot ( Fig. 8b ). This result suggests that β-arrestin-2 is necessary for M3-R to exert its effects on OR-induced cAMP responses in HEK293T cells. 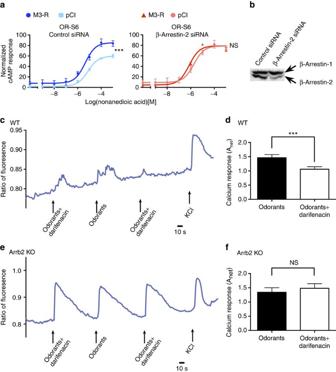Figure 8: β-Arrestin-2 depletion reduces potentiation on OR-mediated cAMP response by M3-R. (a) In HEK293T cells, with control siRNA transfection, M3-R significantly potentiated the cAMP response of OR (left, two-way ANOVA,P<10−4). With β-arrestin-2 siRNA transfection, the potentiation is diminished (right, two-way ANOVA,P=0.63).n=3, error bars indicate standard errors. (b) Efficiency of β-arrestin-2 siRNA in HEK293T cells shown by western blot. (c) A single cell from a β-arrestin-2+/+mouse was stimulated by a mixture of 10 odorants each at 10 μM with or without 0.1 μM darifenacin. The Ca2+signals were monitored as fluorometric ratios (Fura-2 340 nm/380 nm). KCl serves as a positive control. (d) Darifenacin significantly reduced odour-induced Ca2+signals (P=0.0006, two-tailed pairedt-test,n=116 pairs). (e) A single cell from a β-arrestin-2−/−mouse was stimulated by a mixture of 10 odorants each at 10 μM with or without 0.1 μM darifenacin. (f) Darifenacin failed to attenuate odour-mediated responses of OSNs from M3-R−/−mice (P=0.512, two-tailed pairedt-test,n=90 pairs). ***P<0.001. NS, not significant. Figure 8: β-Arrestin-2 depletion reduces potentiation on OR-mediated cAMP response by M3-R. ( a ) In HEK293T cells, with control siRNA transfection, M3-R significantly potentiated the cAMP response of OR (left, two-way ANOVA, P <10 −4 ). With β-arrestin-2 siRNA transfection, the potentiation is diminished (right, two-way ANOVA, P =0.63). n =3, error bars indicate standard errors. ( b ) Efficiency of β-arrestin-2 siRNA in HEK293T cells shown by western blot. ( c ) A single cell from a β-arrestin-2 +/+ mouse was stimulated by a mixture of 10 odorants each at 10 μM with or without 0.1 μM darifenacin. The Ca 2+ signals were monitored as fluorometric ratios (Fura-2 340 nm/380 nm). KCl serves as a positive control. ( d ) Darifenacin significantly reduced odour-induced Ca 2+ signals ( P =0.0006, two-tailed paired t -test, n =116 pairs). ( e ) A single cell from a β-arrestin-2 −/− mouse was stimulated by a mixture of 10 odorants each at 10 μM with or without 0.1 μM darifenacin. ( f ) Darifenacin failed to attenuate odour-mediated responses of OSNs from M3-R −/− mice ( P =0.512, two-tailed paired t -test, n =90 pairs). *** P <0.001. NS, not significant. Full size image To determine whether this model is conserved in OSNs, we tested whether the attenuation of OR activity by M3-R-selective antagonists would also be diminished in OSNs lacking β-arrestin-2. We performed Ca 2+ imaging on acutely dissociated OSNs isolated from either β-arrestin-2 KO (Arrb2 −/− ) or age-matched WT control (Arrb2 +/+ ) mice, stimulated by a mixture of 10 odorants in the presence or absence of 0.1 μM darifenacin. While the Ca 2+ responses in Arrb2 +/+ OSNs were attenuated by darifenacin ( Fig. 8c,d , P =0.0006, two-tailed paired t -test, n =116 pairs), no significant change was observed in OSNs from Arrb2 −/− mice ( Fig. 8e,f , P =0.512, two-tailed paired t -test, n =90 pairs). As the attenuation of OR-mediated Ca 2+ responses by darifenacin was abolished in the absence of β-arretin-2, these findings strongly support our model in which M3-Rs’ effects on OR activity are mediated through inhibition of β-arrestin-2 recruitment. M3-R and ORs do not directly compete for β-arrestin-2 binding To investigate the mechanism by which M3-Rs inhibit β-arrestin-2 recruitment to activated ORs, we asked whether activated M3-Rs directly compete with ORs for β-arrestin-2. This hypothesis leads to the following two predictions: (1) the inhibition of β-arrestin-2 recruitment at ORs by M3-R would be diminished as the amount of β-arrestin-2 expressed increases to exceed a rate-limiting level; (2) ORs would also potentiate the responses of M3-Rs. To test the first prediction, we measured the recruitment of β-arrestin-2 to ORs in HEK293T transfected with ORs, either M3-Rs or M2-Rs, and increasing concentrations of Arrb2-CLuc (Luc-tagged β-arrestin-2). In both ORs tested, OR-S6 and Olfr62, overexpressing Arrb2-CLuc (100 ng per well) did not abolish the inhibition of β-arrestin-2 recruitment by M3-Rs ( Fig. 9a , P <10–4 for both ORs, two-way analysis of variance (ANOVA)), as compared with normal assay conditions (20 ng Arrb2-CLuc cotransfection, P <10 −4 for both ORs, two-way ANOVA). In addition, we tested OR activation under β-arrestin-2 overexpression conditions with and without M3-Rs. While OR activation was reduced by ~95% when β-arrestin-2 was overexpressed (100 ng per well), consistent with the important role of β-arrestin-2 in OR inactivation, the relative fold enhancement of the OR response by M3-R coexpression was stable in all β-arrestin-2 overexpression conditions (1–100 ng per well; Fig. 9b ). To test the second prediction, we compared the Gq-coupled Ca 2+ responses of M3-Rs following carbachol stimulation with and without the coexpression of OR-S6. We did not observe significant changes in M3-Rs response to its own ligand ( Fig. 9c , P =0.856. two-way ANOVA). From these results, we conclude that the ability of M3-Rs to decrease β-arrestin-2 recruitment of ORs is unlikely to be explained by a direct competition for β-arrestin-2 between these two receptors. 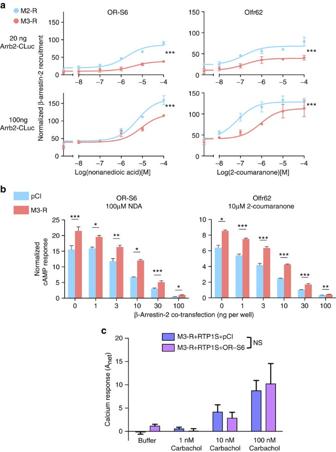Figure 9: The modulation of OR activation by M3-R is not a result of direct competition for β-arrestin-2. (a) The effect of M3-R on β-arrestin-2 recruitment of OR-S6 and Olfr62 with the cotransfection of 20 ng (normal assay condition) or 100 ng (overexpression) Arrb2-CLuc. Coexpression of M3-Rs significantly decreased β-arrestin-2 recruitment of both ORs under normal assay conditions and with Arrb2-CLuc overexpression (two-way ANOVA,P<10−4in all instances) as compared with the control M2-R. (b) cAMP responses of OR-S6 and Olfr62 stimulated by their cognate ligands (100 μM nonanedioic acid and 10 μM 2-coumaranone, respectively). Cells were cotransfected with different amount of β-arrestin-2 (0–100 ng per well) in the presence and absence of M3-Rs. With all the β-arrestin-2 cotransfection amounts, M3-R significantly potentiated the cAMP responses of both ORs (*P<0.05, **P<0.01, ***P<0.001, two-tailedt-test). (c) Ca2+response of M3-Rs to carbachol with and without the coexpression of OR-S6. OR-S6 does not significantly potentiate the response of M3-Rs to carbachol (two-way ANOVA,P=0.856).n=3, error bars indicate standard errors. NS, not significant. Figure 9: The modulation of OR activation by M3-R is not a result of direct competition for β-arrestin-2. ( a ) The effect of M3-R on β-arrestin-2 recruitment of OR-S6 and Olfr62 with the cotransfection of 20 ng (normal assay condition) or 100 ng (overexpression) Arrb2-CLuc. Coexpression of M3-Rs significantly decreased β-arrestin-2 recruitment of both ORs under normal assay conditions and with Arrb2-CLuc overexpression (two-way ANOVA, P <10 −4 in all instances) as compared with the control M2-R. ( b ) cAMP responses of OR-S6 and Olfr62 stimulated by their cognate ligands (100 μM nonanedioic acid and 10 μM 2-coumaranone, respectively). Cells were cotransfected with different amount of β-arrestin-2 (0–100 ng per well) in the presence and absence of M3-Rs. With all the β-arrestin-2 cotransfection amounts, M3-R significantly potentiated the cAMP responses of both ORs (* P <0.05, ** P <0.01, *** P <0.001, two-tailed t -test). ( c ) Ca 2+ response of M3-Rs to carbachol with and without the coexpression of OR-S6. OR-S6 does not significantly potentiate the response of M3-Rs to carbachol (two-way ANOVA, P =0.856). n =3, error bars indicate standard errors. NS, not significant. Full size image The third intracellular loop of M3-R is important for OR modulation Another possible mechanism by which M3-R may inhibit β-arrestin-2 recruitment to activated ORs may be via a direct physical interaction at the receptor and/or G-protein level, as supported by previous data showing that M3-Rs and ORs coimmunoprecipitate in vitro , as well as the fact that downstream M3-R signalling appears to be unimportant for OR activation. One question of interest is whether the interaction between M3-Rs and ORs can be further enhanced by the activation of either receptor, although the interaction is observed in the absence of stimulation [21] . To address this question, we used the split-luciferase system to monitor the interaction between M3-Rs and ORs following their activation. Interestingly, we observed a small yet significant decrease in luciferase signals following the activation of M3-Rs or ORs ( Supplementary Fig. 5 ), suggesting that the interaction between M3-Rs and ORs is not enhanced by receptor activation; the decrement in the split-luciferase signal likely reflects conformational changes within the receptors. If M3-Rs directly potentiates OR activity, we expect that specific functional domains of M3-R would be critical for its interaction with ORs and/or β-arrestin-2. The long third intracellular loop (i3) is the most divergent domain among the muscarinic receptor family members, and is important for M3-R function [33] , [34] , [35] , [36] . We hypothesized that the i3 loop may be necessary for the ability of M3-R to inhibit β-arrestin-2 recruitment of ORs. To test this hypothesis, we interchanged the entire i3 loop of M3-R with that of M2-R and examined how the two resulting chimeric muscarinic receptors modulate OR function. M3-M2L refers to the chimeric M3-R with its i3 loop replaced by that of M2-R, whereas M2-M3L refers to the chimeric M2-R with its i3 loop replaced by that of M3-R ( Fig. 10a ). Interestingly, we found that M3-M2L behaved like M2-R and was unable to inhibit β-arrestin-2 recruitment to ORs. In contrast, M2-M3L decreased β-arrestin-2 recruitment to ORs, mimicking the effect of M3-R ( P <0.0001 for M2 versus M3, M2 versus M2-M3L, M3 versus M3-M2L and M2-M3L versus M3-M2L, two-way ANOVA; Fig. 10b , left). Consistently, M2-M3L, similar to the native M3-R, potentiates OR-mediated cAMP responses, while M3-M2L does not ( P <0.001 for M2 versus M3, M2 versus M2-M3L, M3 versus M3-M2L and M2-M3L versus M3-M2L, two-way ANOVA; Fig. 10b , right). Taken together, these results indicate that the i3 loop of M3-R is necessary and sufficient for M3-Rs to inhibit β-arrestin-2 recruitment and potentiate cAMP responses of ORs upon activation, thereby lending further support to our model ( Fig. 10c ). 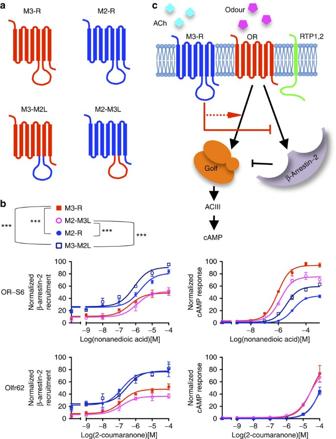Figure 10: The third intracellular loop of M3-R is important for OR potentiation. (a) Chimera construction. The third intracellular loop of M2-R and M3-R were exchanged to generate the following two chimeras: M2-M3L, the chimeric M2-R with the i3 loop replaced by that of M3-R, and M3-M2L, the M3-R with its i3 loop replaced by that of M2-R. (b) β-Arrestin-2 recruitment and cAMP response of two ORs with the coexpression of M2, M3 or chimeras. For both ORs, M3-M2L showed less blocking of β-arrestin-2 recruitment to OR as compared with M3-R. In contrast, M2-M3L showed marked blocking of β-arrestin-2 recruitment. For both ORs, M2-M3L showed substantial potentiation on OR-mediated cAMP responses. ***P<0.01. Two-way ANOVA for β-arrestin-2 recruitment comparisons: OR-S6, M3 versus M2 (P<0.0001), M3 versus M3-M2L (P<0.0001), M2 versus M2-M3L (P<0.0001), M2-M3L versus M3-M2L (P<0.0001); Olfr62, M3 versus M2 (P<0.0001), M3 versus M3-M2L (P<0.0001), M2 versus M2-M3L (P<0.0001), M2-M3L versus M3-M2L (P<0.0001). Two-way ANOVA for cAMP response comparisons: OR-S6, M3 versus M2 (P<0.0001), M3 versus M3-M2L (P<0.0001), M2 versus M2-M3L (P<0.0001), M2-M3L versus M3-M2L (P<0.0001); Olfr62, M3 versus M2 (P=0.002), M3 versus M3-M2L (P=0.001), M2 versus M2-M3L (P<0.0001), M2-M3L versus M3-M2L (P<0.0001).n=3, error bars indicate standard errors. (c) Model for how M3-Rs potentiates OR activation. M3-Rs physically interacts with the OR. The third intracellular loop (i3) of M3-R is important for M3-Rs to inhibit β-arrestin-2 recruitment to activated ORs, and this inhibition is enhanced in the presence of M3-R agonists such as, for example, acetylcholine (ACh). Through the inhibition of β-arrestin-2 recruitment at ORs, M3-R promotes G-protein coupling of ORs and augments OR activation. Figure 10: The third intracellular loop of M3-R is important for OR potentiation. ( a ) Chimera construction. The third intracellular loop of M2-R and M3-R were exchanged to generate the following two chimeras: M2-M3L, the chimeric M2-R with the i3 loop replaced by that of M3-R, and M3-M2L, the M3-R with its i3 loop replaced by that of M2-R. ( b ) β-Arrestin-2 recruitment and cAMP response of two ORs with the coexpression of M2, M3 or chimeras. For both ORs, M3-M2L showed less blocking of β-arrestin-2 recruitment to OR as compared with M3-R. In contrast, M2-M3L showed marked blocking of β-arrestin-2 recruitment. For both ORs, M2-M3L showed substantial potentiation on OR-mediated cAMP responses. *** P <0.01. Two-way ANOVA for β-arrestin-2 recruitment comparisons: OR-S6, M3 versus M2 ( P <0.0001), M3 versus M3-M2L ( P <0.0001), M2 versus M2-M3L ( P <0.0001), M2-M3L versus M3-M2L ( P <0.0001); Olfr62, M3 versus M2 ( P <0.0001), M3 versus M3-M2L ( P <0.0001), M2 versus M2-M3L ( P <0.0001), M2-M3L versus M3-M2L ( P <0.0001). Two-way ANOVA for cAMP response comparisons: OR-S6, M3 versus M2 ( P <0.0001), M3 versus M3-M2L ( P <0.0001), M2 versus M2-M3L ( P <0.0001), M2-M3L versus M3-M2L ( P <0.0001); Olfr62, M3 versus M2 ( P =0.002), M3 versus M3-M2L ( P =0.001), M2 versus M2-M3L ( P <0.0001), M2-M3L versus M3-M2L ( P <0.0001). n =3, error bars indicate standard errors. ( c ) Model for how M3-Rs potentiates OR activation. M3-Rs physically interacts with the OR. The third intracellular loop (i3) of M3-R is important for M3-Rs to inhibit β-arrestin-2 recruitment to activated ORs, and this inhibition is enhanced in the presence of M3-R agonists such as, for example, acetylcholine (ACh). Through the inhibition of β-arrestin-2 recruitment at ORs, M3-R promotes G-protein coupling of ORs and augments OR activation. Full size image Here, we extensively characterized the mechanisms by which M3-Rs can modulate OR activation in native OSNs and heterologous cells by using Ca 2+ imaging, electrophysiological, pharmacological and genetic tools. Further, we developed a novel assay to assess β-arrestin-2 recruitment to elucidate the molecular mechanism by which M3-Rs exert action on OR activation. We confirmed that M3-Rs are expressed in the cilia layer of the OE and showed that the genetic ablation of M3-Rs does not affect the anatomical organization of the OE nor the development of olfactory cilia ( Fig. 1 and Supplementary Fig. 1 ). We then demonstrated that darifenacin, a selective antagonist for M3-R, significantly attenuates odour-induced Ca 2+ and electrical signals in OSNs from WT, but not from M3-R KO mice ( Figs 2 and 3 ). Moreover, carbachol and acetylcholine enhanced odour-induced transduction currents in OSNs from WT animals ( Fig. 4 ). These data strongly support a role for acetylcholine in modulating the sense of smell at the periphery. Furthermore, we investigated the molecular mechanism underlying this cholinergic modulation. Our results support a model in which M3-Rs amplifies OR activity by blocking the interaction between β-arrestin-2 and ORs. Consistent with this model, depleting β-arrestin-2 in both heterologous cells and OSNs almost completely abolishes the potentiation of ORs by M3-Rs. The dynamic regulation of β-arrestin-2-mediated recruitment of ORs by M3-Rs, along with the clear potentiation of this effect in the presence of M3-R ligands, suggests a potential pathway through which olfactory perception can be modulated by cholinergic signalling at the periphery. M3-R was first identified as a non-OR GPCR that modulates OR activity through a screen for candidate proteins that potentiate OR activation in HEK293T cells. The M3-R transcript and protein have previously been shown to colocalize with olfactory marker protein-expressing OSNs in the OE. Ogura et al . [17] recently reported that M3-R protein is expressed in the supporting cells, and that acetylcholine suppresses forskolin-induced Ca 2+ increase in OSNs. To address these discrepancies, we used M3-R −/− mice to determine expression patterns of M3-R as well as its modulatory effects on OR function. Our immunostaining results are consistent with the original report showing that M3-R protein is predominantly expressed in the cilia of the OE ( Fig. 1 ), although there is also some weak staining of the supporting cells in some regions. In control experiments without the primary M3-R antibody, we did not observe M3-R staining in the cilia layer, but we did observe similar staining in the supporting cells, suggesting that the staining in the supporting cells may be nonspecific for M3-R. Our data support a model in which M3-Rs potentiate OR activity upstream of type III adenylyl cyclase. This potentiation could overwhelm downstream suppressive effects by acetylcholine. This model could in turn reconcile potentiation of odour-induced OSN activity and the suppression of forskolin-induced activity in some OSNs. Given that M3-Rs are expressed in OSNs, it is plausible that the interaction of M3-Rs and ORs found in HEK293T cells is not purely a result of overexpression, but may be relevant for physiological functions of ORs and, consequently, OSNs. Consistent with the observations made in HEK293T cells transfected with ORs and M3-Rs [21] , pharmacological antagonism of M3-Rs by darifenacin reduced odour-induced responses in OSNs from M3-R +/+ mice ( Figs 2 and 3 ). As expected, the effect of darifenacin was abolished in OSNs from M3-R −/− mice ( Figs 2 and 3 ), further supporting the specificity with which darifanacin acts on M3-Rs in these neurons. In addition, results from our prior in vitro analyses suggest that there is significant OR-dependent heterogeneity in the effect of M3-R expression on OR responses. For some Ors, the effect of M3-R expression is far greater than others. Likewise, during Ca 2+ imaging and patch-clamp analysis, it was clear that there was also variance among OSNs in their responses to darifenacin. We also found that costimulating OSNs with odorants and a muscarinic agonist, carbachol, or the physiological muscarinic ligand acetylcholine, enhanced the odour responses ( Fig. 4 ). Curiously, a small subset of OSNs from WT animals showed the opposite modulation by M3-R antagonists and agonists ( Figs 3c and 4b ). One possibility is that darifenacin has off-target effects and that in the absence of the stronger effect of darifenacin on M3-Rs, M3-R −/− neurons show a nonspecific response to darifenacin. Alternatively, some OSNs may express low levels of the Gi-coupling muscarinic family members, including M2-R and M4R. Although darifenacin is an M3-R-preferring antagonist, it does show significant binding and antagonism with the other muscarinic members [37] . How does M3-R inhibit the recruitment of β-arrestin-2 to ORs? We have shown that the inhibition is not explained by competition for β-arrestin-2 between the two receptors [38] , [39] , [40] , [41] , [42] , [43] , [44] , [45] , [46] , [47] , [48] , [49] , [50] , [51] . In addition, results from our chimeric receptor analysis suggests that the large third intracellular loop of the M3-R is necessary and sufficient for its ability to inhibit the recruitment of β-arrestin-2 to ORs and ultimately, potentiate OR-mediated cAMP responses. However, the mechanism by which M3-R activation represses β-arrestin-2 recruitment to ORs remains to be further elucidated. One possibility is that M3-R-OR heteromerization allosterically inhibits the ability of ORs to bind β-arrestin-2. For example, the binding of M3-Rs to ORs could spatially limit the access of β-arrestin molecules to key binding sites on ORs. Another possibility is that the binding of activated M3-Rs shifts the protein conformation of ORs to lower their β-arrestin-2 affinity. Structural analysis of the OR-M3-R complex will be needed to evaluate this hypothesis. Finally, M3-Rs could act indirectly by regulating the activity of other GPCR interacting proteins, such as GPCR kinases, which mediate the phosphorylation of activated ORs to facilitate β-arrestin recruitment. Although it has been two decades since β-arrestin-2 was shown to participate in OR desensitization, only one OR has ever been reported to recruit β-arrestin-2 in heterologous cells by the use of bioluminescence resonance energy transfer [9] , [10] . Here we describe the first β-arrestin-2 recruitment assay that successfully generates quantitative concentration-dependent readouts for a diverse set of ORs, using a split-luciferase system that has been successfully applied previously to measure β-arrestin recruitment to several activated GPCRs [52] , [53] , [54] , [55] . It has been shown that β-arrestins mediate distinct signalling cascades apart from G-protein-initiated pathways, including MAP kinases ERK1/2, and that biased ligands can preferentially trigger one pathway over the other [13] , [56] , [57] . Interestingly, the odour-stimulated MAP kinase pathway [58] has been shown to enhance the survival of OSNs [59] , although it is unclear if β-arrestin-2 mediates this effect. Our analysis on OR-EG-activating odorants suggests that this ligand bias also exists for ORs [60] , and provides a basis for future studies of OR-mediated β-arrestin signalling. The OE is innervated by parasympathetic nerve endings that release acetylcholine [14] , [15] , [16] , which is active when stress levels are low, for instance, during feeding. Interestingly, M3-R KO mice have been shown to have significantly lower body weight compared with their WT siblings due to unexplained hypophagia. Although we found no gross defect in the OE nor evidence of decreases in the number or health of OSNs by examining the OE in M3-R KOs as compared with their WT littermates, the current study suggests that muscarinic modulation of OSNs may be relevant to odour sensitivity. While it is speculative at this point, it is possible that the role of M3-Rs in appetite regulation and the resultant hypophagia in M3-R KO mice may be, at least in part, a result of decreased olfactory perception. In addition, parasympathetic stimulation also led to secretion of nasal mucus. Under these circumstances, the M3-R/OR interaction may facilitate odour detection or provide a mechanism to compensate for the decreased ability to smell due to hypersecretion. Furthermore, when chemical compounds (usually irritating) stimulate the local acetylcholine-releasing cells in the OE, the acetylcholine released may enhance the sensitivity of OSNs via M3-Rs, which may help the organism to identify the source of stimulation. Animals WT C57/Bl6 mice were purchased from Jackson Laboratory and breeding pairs of heterozygous M3-R KO mice (backcrossed to C57Bl/6 background) were purchased from Taconic (no. 1455; ref. 23 ). β-Arrestin-2 KO and age-matched WT control mice were gifts from Dr Robert Lefkowitz [61] . Genotyping was performed according to the protocol provided by Taconic. Animals of either sex were used at the age of 3–5 weeks. The procedures of animal handling and tissue harvesting were approved by the Institutional Animal Care and Use Committee of the University of Pennsylvania and the Duke University. Patch clamp As described previously (Ma et al . [26] ), mice were deeply anaesthetized by intraperitoneal injection of ketamine and xylazine (200 and 15 mg kg −1 , respectively), and then decapitated. The head was immediately put into icy Ringer’s solution, which contained (in mM) NaCl 124, KCl 3, MgSO 4 1.3, CaCl 2 2, NaHCO 3 26, NaH 2 PO 4 1.25 and glucose 15; pH 7.6 and 305 mOsm. The pH was kept at 7.4 after bubbling with 95% O 2 and 5% CO 2 . From each nostril, the olfactory mucosa attached to the nasal septum and from the dorsal recess was removed en bloc and kept in oxygenated Ringer. Before use, the entire mucosa was peeled away from the underlying bone and transferred to a recording chamber with the mucus layer facing up. While recording, oxygenated Ringer was continuously perfused at 25±2 ˚C. The dendritic knobs of OSNs in intact OE were visualized through an upright microscope (Olympus BX61WI) with a × 40 water-immersion objective. An additional × 4 magnification was achieved by an accessory lens in the light path. Electrophysiological recordings were controlled by an EPC-9 amplifier combined with Pulse software (HEKA Electronic, Germany). Perforated patch clamp was performed on the dendritic knobs by including 260 μM nystatin in the recording pipette, which was filled with the following solution (in mM): KCl 70, KOH 53, methanesulfonic acid 30, EGTA 5.0, HEPES 10 and sucrose 70; pH 7.2 (KOH) and 310 mOsm. Under voltage-clamp mode, the signals were initially filtered at 10 kHz and then at 2.9 kHz. For odour-induced transduction currents, which are relatively slow and long lasting, the signals were sampled at 333 Hz. Further filtering offline at 60 Hz did not change the response kinetics or amplitudes, indicating that the sampling rate was sufficient and that signal aliasing was not a concern. A seven-barrel pipette, placed ~25 μm downstream from the recording site, was used to deliver stimuli by pressure ejection (at 20 psi or 138 kPa) via a picospritzer (Pressure System IIe). The pulse length was kept at 300 ms to ensure that the neurons were stimulated by the intrapipette concentration [62] . The odorant mixture contained 19 odorants at equal molar concentration of 100 μM including: heptanol, octanol, hexanal, heptanal, octanal, heptanoic acid, octanoic acid, cineole, amyl acetate, (+)-limonene, (–)-limonene, (+)-carvone, (–)-carvone, 2-heptanone, anisaldehyde, benzaldehyde, acetophenone, 3-heptanone and Ethyl vanillin. Darifenacin, carbachol and acetylcholine were dissolved in Ringer’s solutions and included in the puffing pipettes. In the antagonist experiments ( Fig. 3 ), individual barrels were filled either with the odorant mixture or with the odorant mixture plus 0.1 μM darifenacin; only one barrel was open for pressure ejection at a time. For the agonist experiments ( Fig. 4 ), because we chose to test multiple agonists, we devised a method to reduce variability in individual barrel opening sizes by modifying the delivery system so that the odorant mixture was always ejected from the same barrel independent of the drug used. The final mixture consisted of odorants in conjunction with a second open barrel filled with Ringer’s solution or one of the three agonist solutions (0.1 μM carbachol, 1 μM carbachol or 1 μM acetylcholine). Consequently, the delivery pressure for each barrel was approximately reduced by half (due to the opening of two barrels at the same time) in the agonist experiments and the control odour responses were smaller than those in the antagonist experiments. All compounds and chemicals were obtained from Sigma-Aldrich. Calcium imaging To measure Ca 2+ levels in acutely dissociated OSNs, we followed a previously described procedure [21] . Dissected adult mouse OE was treated with 0.025% trypsin (Invitrogen) for 12 min at 37 °C. Minced tissues were then ‘printed’ on poly- D -lysine-coated coverslips. Cells were loaded with Fluo-4 (4 μM; Invitrogen) and Fura red (7 μM; Invitrogen) or Fura-2 (5 μM) for 60 min at room temperature. A Leica confocal microscope or A Zeiss AxioObserver 1.0 inverted microscope was used to record Ca 2+ -dependent cell fluorescence. Cells were exposed to a constant flow of bath solution (Hank’s buffer containing 10 mM HEPES). Odorant solution (a mixture of 10 odorants: isoeugenol, vanillin, coumarin, nonanoic acid, heptanal, benzyl acetate, nonanediol, acetophenone, octanol and (−)-carvone at 10 μM each) was applied for ~8 s by changing the bath solution with a peristaltic pump. For data analysis, we first counted neurons by identifying those cells that showed a clear Ca 2+ response to KCl. Of these, cells that showed a response to the odorant mix, to the odorant mix and antagonist, or to both were marked for further analysis. Each field that we recorded typically contained 40–200 KCl-responding cells and 1–5 odour-responding cells. We used Euler’s trapezoidal method to calculate and compare the responses of each cell to the odorant mix with or without antagonist. All data analysis was done with ImageJ, MetaMorph, MetaFluor, Igor Pro and Microsoft Excel. Immunohistochemistry After decapitation, the head was immediately put into 4% paraformaldehyde (Sigma) overnight at 4 °C, and then subject to decalcification in 0.5 M EDTA (pH 8.0) for 2 days. The nose was cut into 20 μm coronal sections on a cryostat. After antigen retrieval in 95 °C water bath for 12 min, nose sections were first blocked for 60 min in TPBS (0.3% Triton X-100 in phosphate-buffered saline) with 2% bovine serum albumin and then incubated at 4 °C with the primary antibodies in the same solution for overnight. Immunofluorescence was achieved by reaction with appropriate secondary antibodies at 1:400 for 1 h. Tissues were washed in TPBS and mounted in Vectashield (Vector Laboratories). Pictures were taken under a Zeiss LSM 510 confocal microscope. The primary antibodies included biotinylated Dolichos biflorus agglutinin (1:300, B-1035, Vector Laboratories) and rabbit anit-M3-R (1:300, M0194, Sigma-Aldrich), and the secondary antibodies included streptavidin conjugate 488 (S-32354, Invitrogen) and donkey-anti-rabbit-568 (A10042, Invitrogen). 4′,6-Diamidino-2-phenylindole, dihydrochloride (D1306, Invitrogen) was used to stain the cell nuclei. DNA and vector preparation The open reading frames were amplified using Phusion polymerase (Finnzymes) following manufacturer’s protocols. Amplified fragments were cloned into pCI (Promega) or Rho-pCI for sequence verification. Unless otherwise noted, ORs were cloned into Rho-pCI to introduce a Rho-tag (first 20 amino acids of rhodopsin) at the N-termini. The Rho-tag is known to facilitate the heterologous expression of ORs [63] . Primer sequences for split-luciferase constructs are available in Supplementary Methods . Cell culture HEK293T cells were maintained in minimal essential medium containing 10% fetal bovine serum with penicillin–streptomycin and amphotericin B at 37 °C and 5% CO 2 . Split-luciferase assay The construction of split-luciferase plasmids was as described by Luker et al . [28] with modifications. Briefly, the N- and C-terminal fragments of firefly luciferase (NLuc and CLuc) were fused by chimeric PCR to the C-termini of ORs and β-arrestin-2, respectively, connected by a flexible Gly/Ser linker. The chimeric fragments were cloned into Rho-pCI (ORs) or pCI (β-arrestin-2) between the MluI and NotI sites. See Supplementary Methods for details. The primary antibodies used to characterize the fusion proteins include mouse anti-rhodopsin 4D2 (1:200, provided by R. Molday), rabbit anti-β-arrestin A1CT (1:3,000, provided by R. Lefkowitz) and goat anti-luciferase (1:1,000, G7451, Promega). For split-luciferase assay, cells were seeded on poly- D -lysine-coated 96-well plates (Nunc). Twenty-four hours after seeding, cells were transfected with various combination of split-luciferase constructs using Lipofectamine 2000 (Invitrogen) following manufacturer’s protocols. Twenty-four hours after transfection, cells were rinsed by 50 μl of HBSS (Hank's Balanced Salt Solution, Invitrogen) containing 10 mM HEPES and 1 mM glucose (loading buffer). Cells were then loaded with 25 μl 2% GloSensor reagent (Promega) dissolved in loading buffer for 2 h at room temperature. After loading, cells were stimulated with odorants and incubated at 37 °C and 5% CO 2 for 3–6 h. Photon counts were then measured with a plate reader (BMG Labtech) at bioluminescence mode. A stably expressed Renilla luciferase (pRL-SV40, Promega) was cotransfected as an internal control. Normalized split-luciferase activity was calculated by the formula: (L N −L Max )/(L MAX −L MIN ), where L MAX and L MIN are the maximum and minimum luciferase value on the plate or a set of plates. The data were analysed using GraphPad Prism 5. Dual-Glo assay The Dual-Glo assay for ORs was as described previously [64] . Briefly, HEK293T cells were plated on 96-well plates. Eighteen to 24 h after plating, cells were transfected with plasmids coding for OR, RTP1S, CRE-luciferase and pRL-SV40. Eighteen to 24 h later, cells were stimulated by incubation with odorants in CD293 for 4 h at 37 °C and 5% CO 2 to allow for CRE-luciferase expression. Luciferase and Renilla luciferase activities were measured using Dual-Glo kit following manufacturer’s protocols (Promega). Normalized luciferase activity was calculated by the formula (L N −L Max )/(L MAX −L MIN ), where L MAX and L MIN are the maximum and minimum luciferase value on the plate or a set of plates. Data was analysed using GraphPad Prism 5. PLC inhibitors PLC active inhibitor U73122 was purchased from Sigma. For Dual-Glo luciferase assays, the drug was coadministered simultaneously with odorants. siRNA depletion of β-arrestin-2 Double-strand interfering RNA targeting β-arrestin-2 and control were as described by Ahn et al . [32] HEK293T cells were maintained as described above. For siRNA transfection, cells were plated on six-well plates. Twenty-four after plating, β-arrestin-2 or control siRNAs (Dharmacon, Thermo Scientific) were transfected using GeneSilencer (Genlantis) following manufacturer’s protocols. The knockdown was allowed for more than 48 h before cells were re-plated on 96-well plates for Dual-Glo assay. The knockdown efficiency was confirmed by western blot. Generation of M3-M2 chimeras To generate chimeric receptors of M3-R and M2-R, we interchanged the entire i3 loop of M3-R and M2-R by the use of PCR-based mutagenesis using chimeric primers that contain regions of both receptors. For example for the M3-M2L (where the entire i3 loop of M3-R was replaced with that of M2-R), the first set of primers targeted the region upstream of the i3 domain with 18–20 bp matching to the M3-R and 18–20 bp matching the M2-R. Then, two separate PCRs were used to amplify either the upstream region from M3-R or the downstream region from M2-R. The two linear products were then combined along with generic vector primers to amplify the self-primed fusion products. This creates a chimera that has only the M3-R sequences upstream of the i3 loop site, and only M2-R sequences form the i3 loop site downstream. Next, the process was repeated with a second set of internal chimeric primers, except these chimeric primers targeted the downstream region of the i3 loop using the M3-M2 chimera generated in the first step. More details can be found in ref. 65 . Statistical analysis Fisher’s exact test and two-way ANOVA were performed using the GraphPad Prism. Student’s t -test was performed using the built-in function in Excel. Average is shown as mean±standard errors. How to cite this article: Jiang, Y. et al . Muscarinic acetylcholine receptor M3 modulates odorant receptor activity via inhibition of β-arrestin-2 recruitment. Nat. Commun. 6:6448 doi: 10.1038/ncomms7448 (2015).